Near-ideal theoretical strength in gold nanowires containing angstrom scale twins Although nanoscale twinning is an effective means to enhance yield strength and tensile ductility in metals, nanotwinned metals generally fail well below their theoretical strength limit due to heterogeneous dislocation nucleation from boundaries or surface imperfections. Here we show that Au nanowires containing angstrom-scaled twins (0.7 nm in thickness) exhibit tensile strengths up to 3.12 GPa, near the ideal limit, with a remarkable ductile-to-brittle transition with decreasing twin size. This is opposite to the behaviour of metallic nanowires with lower-density twins reported thus far. Ultrahigh-density twins (twin thickness<2.8 nm) are shown to give rise to homogeneous dislocation nucleation and plastic shear localization, contrasting with the heterogeneous slip mechanism observed in single-crystalline or low-density-twinned nanowires. The twin size dependent dislocation nucleation and deformation represent a new type of size effect distinct from the sample size effects described previously. The device integration of Au nanowires (NWs) hinges upon better understanding the ultrahigh strength [1] and fracture behaviour of individual NWs under nanoscale deformation by direct measurements. As a model material, bulk Au is intrinsically the most ductile and malleable metal with a tensile ductility in the range of 0.2~0.4 (ref. 2 ). Past experimental studies showed that Au NWs can be pulled with a strain up to 50% (ref. 3 ), and long atomic chains can be formed until the last atomic bond breaks [4] . Recent experiments and molecular dynamics (MD) simulations also showed that sub-10 nm-sized Au single crystals possess very good ductility before fracture [5] , [6] . However, it was also reported in another recent study that ultrathin Au NWs can fail via brittle fracture with negligible ductility [7] . Brittle failure was attributed to deformation twinning [7] , whereas this mechanism is recognized as promoting superplastic deformation in metallic NWs [3] , [8] , [9] . In view of these conflicting observations, one question naturally arises: how to decisively control fracture in metallic NWs? The plastic deformation and fracture of bulk ultrafine-grained metals containing nanoscale twins has been extensively studied since first being observed 8 years ago [10] . It is now well-established that nanotwinned face-centred-cubic (FCC) metals have superior mechanical strength, remarkably high ductility, and better tolerance to fatigue crack initiation with decreasing twin thickness ( λ ) [11] , [12] , [13] . Below a specific limit ( λ <15 nm), reducing λ dramatically enhances ductility due to softening effects, attributed to heterogeneous nucleation and propagation of partial dislocations at the intersection of pre-existing twin boundaries (TBs) with grain boundaries (GBs) [11] , [12] , [14] . Likewise, in FCC single-crystalline NWs without GBs, heterogeneous nucleation of new partial dislocations from free surfaces is prominent [5] , [6] , [15] . Moreover, introducing low-density twins (LDTs) to single-crystalline NWs can give rise to extensive strain-hardening and plastic flow after yielding, owing to the blockage of partial slip by TBs [5] , [15] . However, the maximum strength achieved in such materials is still considerably smaller than the ideal strength, which theoretically refers to the stress at elastic instability in a defect-free infinite crystal [15] . Furthermore, although ultrahigh-density twins (UDTs) are frequently observed in metallic NWs synthesized chemically [16] , [17] , [18] , deformation and failure in NWs with growth UDTs remain largely unexplored, specifically near the minimum limit of twin size (that is λ =0.7 nm). Here we present a series of in-situ tensile tests on Au NWs with UDTs conducted under transmission electron microscopy (TEM)-atomic force microscopy (AFM), as well as a detailed description of underlying mechanisms of deformation by high-resolution TEM (HRTEM) combined with MD computer simulations. We show that UDTs provoke a ductile-to-brittle transition at a critical size ( λ =2.8 nm), controlled by homogeneous nucleation of dislocations inside the NWs followed by shear localization and confined microplasticity at TBs. This new regime turns ultrathin Au NWs into brittle-like materials with near-ideal strength, and is unlike the heterogeneous nucleation of partial slip from free surfaces that has commonly been reported for Au NWs with no twins and LDTs. 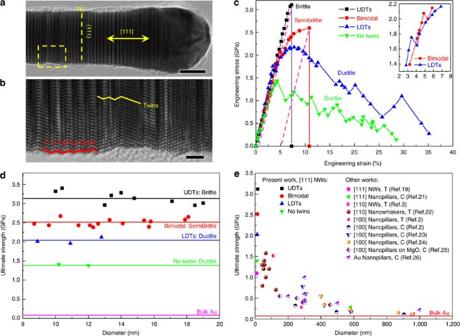Figure 1: Microstructure and mechanical properties of ultra-twinned Au NWs. (a) Morphology of as-synthesized Au NW. Scale bar, 10 nm. (b) High-resolution TEM (HRTEM) image of the yellow-boxed area inashows UDTs distributed along the NW axis ranging from three atomic layers (0.7 nm) to a few nanometres. {111} microfaceting can also be observed at the free surface. Scale bar, 2 nm. (c) Representative stress–strain curves for Au NWs with different structures obtained byin-situTEM–AFM experiments. Dash lines in pink colour indicate the permanent inelastic deformation after fracture. The diameter of samples with either UDTs or bimodal structures are almost identical, 14.5 and 13.4 nm respectively. The inset shows a close-up view of the yield points in the specimens with bimodal and LDTs. (d) Strength distribution in Au NWs with different fracture modes tested in this study. (e) Comparison of ultimate strengths in Au nanocrystals deformed by tension (T) or compression (C) experiments. The flow stress at 10% strain is used as the ultimate strength of compression tests on nanopillars. In-situ mechanical measurements in Au NWs Figure 1 presents the microstructure of ultra-twinned Au NWs as synthesized in this study, along with mechanical properties of these materials under pure tensile loading. The growth direction of Au NWs is along <111> ( Fig. 1a ), with the diameter between 8 and 20 nm. Detailed TEM analysis reveals that parallel UDTs are perpendicular to the wire axis, and that the NW surface is made of {111} microfacets ( Fig. 1b ). Supplementary Fig. S1 shows the twin distributions in two types of Au NWs exhibiting distinct mechanical behaviour. The first type represents NWs with UDTs, in which λ varies over a narrow range from three atomic layers ( λ =0.7 nm) to ~2 nm ( Supplementary Fig. S1a ). In the second type, the NWs show a bimodal twin distribution with a mixture of UDT and LDT spacings ( Supplementary Fig. S1b ). Also, we note that slight departure from the <110> zone axis could make some of the UDTs invisible ( Supplementary Fig. S2 ). Figure 1: Microstructure and mechanical properties of ultra-twinned Au NWs. ( a ) Morphology of as-synthesized Au NW. Scale bar, 10 nm. ( b ) High-resolution TEM (HRTEM) image of the yellow-boxed area in a shows UDTs distributed along the NW axis ranging from three atomic layers (0.7 nm) to a few nanometres. {111} microfaceting can also be observed at the free surface. Scale bar, 2 nm. ( c ) Representative stress–strain curves for Au NWs with different structures obtained by in-situ TEM–AFM experiments. Dash lines in pink colour indicate the permanent inelastic deformation after fracture. The diameter of samples with either UDTs or bimodal structures are almost identical, 14.5 and 13.4 nm respectively. The inset shows a close-up view of the yield points in the specimens with bimodal and LDTs. ( d ) Strength distribution in Au NWs with different fracture modes tested in this study. ( e ) Comparison of ultimate strengths in Au nanocrystals deformed by tension (T) or compression (C) experiments. The flow stress at 10% strain is used as the ultimate strength of compression tests on nanopillars. Full size image Figure 1c shows that the mechanical response of Au NWs with UDTs differs markedly from that of Au NWs with LDTs and no twins. The ultimate strength of Au NWs with no twins was found equal to 1.43 GPa with no strain-hardening after yielding, in excellent agreement with past experimental measurements in pure single-crystalline Au NWs [19] . This value is >30 times higher than the tensile strength of micrometre-thick polycrystalline Au films, which is typical due to plasticity size effects [20] . The mechanical response of Au NWs with LDTs is characterized by significant strain-hardening with an ultimate strength of ~2.05 GPa after yielding (~1.7 GPa), as well as by a sizeable ductility (~35%). Figure 1c shows that this behaviour contrasts with that of Au NWs with UDTs where strain-hardening is found to disappear, ductility is considerably reduced, and the elastic limit increases to ~3.12 GPa ( Fig. 1c ), which is much higher than that of our Au NWs with LDTs and no twins ( Fig. 1d ) and single-crystalline Au nanocrystals reported in the literature [2] , [3] , [19] , [21] , [22] , [23] , [24] , [25] , [26] ( Fig. 1e ). Remarkably, this limit corresponds to a critical resolved shear stress of 0.98 GPa for partial {111}<112> slip (Schmid factor=0.314), which is very close to the ideal shear strength of 1.42 GPa for pure Au reported from past first-principle calculations [27] . Moreover, the fracture behaviour of Au NWs with UDTs is brittle-like with a flat fracture surface perpendicular to the loading axis ( Supplementary Fig. S3a ). Although the total elongation is about 7.2% due to the high elastic strain, plastic elongation at failure is negligible (<1%). In contrast, the behaviour of NWs with bimodal structure appears to be semibrittle with slightly lower yield strength (~2.1 GPa) and limited, but finite inelastic deformation (~5%) and strain-hardening up to ~2.52 GPa ( Fig. 1c ). For both brittle and semibrittle fracture modes, no apparent plasticity is observed away from the fracture zone, but an interesting feature is that a tiny tip is formed on the failure surface in semibrittle NWs only ( Supplementary Fig. S3b ). Homogeneous dislocation nucleation and deformation The above results enable us to conclude that a sharp transition from ductile plasticity to brittle fracture takes place in ultra-twinned Au NWs with increasing twin density. The nature of the ductile-to-brittle transition is further examined by in-situ HRTEM and MD computer simulations. First, we consider the deformation and fracture of Au NWs with LDTs and no twins. 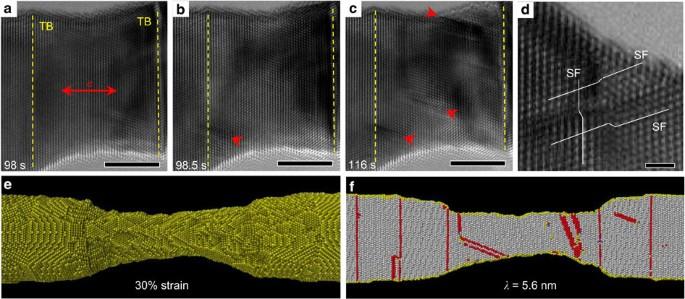Figure 2: Heterogeneous dislocation nucleation in Au NWs with LDTs (λ>5.6 nm). (a) TEM image of an Au NW with LDTs. TBs are marked out by a dash line in yellow colour. Scale bar, 5 nm. (b,c) During tensile loading, partial dislocations with SFs nucleate heterogeneously from the free surface, propagate and are blocked by the TBs, as marked out by the red arrows. Scale bar, 5 nm. (d) Interaction of surface dislocations on different {111} slip planes to form SF cross-structures from a different NW withλ~10 nm. Scale bar, 1 nm. (e) Full atomistic view and (f) cross-sectional view of a NW with uniform twin distribution andλ=5.6 nm at 30% tensile strain as modelled by MD simulation. The colour coding corresponds to surface atoms in yellow colour, atoms in TBs and SFs in red colour, and atoms in perfect FCC crystal arrangement in grey colour. Figure 2a–c and Supplementary Fig. S4 confirm that the deformation of Au NWs with LDTs and no twins is dominated by dislocations nucleated from free surfaces [5] , [6] , [15] . In the Au NWs with LDTs, uniform plastic elongation followed by necking primarily occurs between TBs with the largest λ ( Supplementary Fig. S4a–c and Supplementary Movie 1 ). TBs are also found to act as barriers for partial dislocation motion ( Fig. 2b ), thus contributing to the observed strengthening and strain-hardening effects [5] , [11] , [15] . Interestingly, stacking faults (SFs) nucleated on different {111} planes interact to form SF cross-structures ( Fig. 2d ), which coincides well with the SF structure shown in Fig. 2f when a NW with λ =5.6 nm and a uniform twin distribution is strained in tension by MD simulation. Similarly, the MD simulations show extensive plastic deformation mediated by partial dislocations with SFs nucleated from the surface ( Fig. 2e ), uniform elongation between two TBs ( Supplementary Movie 2 ), and typical ductile stress–strain curves ( Supplementary Fig. S5 ) when λ is as small as 5.6 nm. Figure 2: Heterogeneous dislocation nucleation in Au NWs with LDTs ( λ >5.6 nm). ( a ) TEM image of an Au NW with LDTs. TBs are marked out by a dash line in yellow colour. Scale bar, 5 nm. ( b , c ) During tensile loading, partial dislocations with SFs nucleate heterogeneously from the free surface, propagate and are blocked by the TBs, as marked out by the red arrows. Scale bar, 5 nm. ( d ) Interaction of surface dislocations on different {111} slip planes to form SF cross-structures from a different NW with λ ~10 nm. Scale bar, 1 nm. ( e ) Full atomistic view and ( f ) cross-sectional view of a NW with uniform twin distribution and λ =5.6 nm at 30% tensile strain as modelled by MD simulation. The colour coding corresponds to surface atoms in yellow colour, atoms in TBs and SFs in red colour, and atoms in perfect FCC crystal arrangement in grey colour. Full size image The fracture of a brittle-like NW with UDTs is displayed in Fig. 3 for comparison. In this example, the twin thickness λ is less than 2.1 nm with a predominance of twins at the minimum limit of 0.7 nm ( Supplementary Fig. S1a ). Under tension, the NW first experiences considerable elastic elongation as evidenced by the space increase between TB 3 and TB 4 in Fig. 3b , but sudden failure occurs at an applied strain of 6.8% ( Fig. 3c–e and Supplementary Movie 3 ). The fracture process is materialized over such a short timescale that rare dislocation activity is observed, which is at odds with the larger slip deformation and ductility observed in single-crystalline twin-free Au NWs [3] , [6] and Au NWs with LDTs. However, the grains formed in the fractured tips ( Fig. 3d ) indicate that significant slip and de-twinning have occurred in the confined zone separating TB 1 and TB 4 . This result is further supported by the MD simulations where a net reduction in ductility and shift to brittle-like fracture are manifest in NWs with a {111}-microfaceted surface structure and λ ≤2.8 nm ( Supplementary Fig. S5 ), although the ductile-to-brittle transition seems less pronounced if NWs are modelled with a perfectly circular shape ( Supplementary Fig. S6 ). Moreover, the simulated fracture is contained within a short NW segment exhibiting significant de-twinning ( Fig. 3f ) as in the TEM experiments. A salient feature in MD simulations is that the onset of yielding in brittle-like NWs proves to be controlled by homogeneous nucleation of dislocations between TBs ( Fig. 3h ), as opposed to heterogeneous deformation from free surfaces ( Fig. 2a–c ). 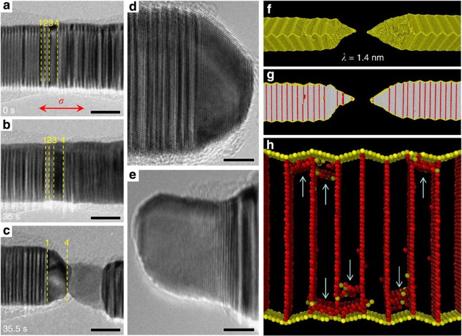Figure 3: Tensile deformation and fracture in brittle-like Au NWs with UDTs (λ<2.8 nm). (a) TEM image of a pristine Au NW showing UDTs ranging from 0.7–2.1 nm, viewed in [110] zone axis. Twin interfaces of interest in the fracture zone are marked as TB1—TB4. Scale bar, 10 nm. (b) Under tensile loading, the NW experiences elastic elongation as evidenced by the increase in spacing between TB3and TB4. Scale bar, 10 nm. (c) At the elastic strain of 6.8%, the Au NW breaks suddenly with a relatively flat fracture surface, typically encountered in brittle fracture. Scale bar, 10 nm. (d,e) Post-deformation fracture morphology of Au NWs at the two ends. A large de-twinned grain is found at both ends. Scale bar, 5 nm. (f) Full atomistic view and (g) cross-sectional view of Au NW with uniform twin distribution andλ=1.4 nm after fracture at 5.5% tensile strain by MD simulation. (h) Close-up view of the fracture region at the onset of yielding showing the homogeneous nucleation of dislocations indicated by vertical arrows, near surface facets but inside the NW. Atoms in perfect FCC crystal arrangement have been omitted for clarity. Figure 3: Tensile deformation and fracture in brittle-like Au NWs with UDTs ( λ <2.8 nm). ( a ) TEM image of a pristine Au NW showing UDTs ranging from 0.7–2.1 nm, viewed in [110] zone axis. Twin interfaces of interest in the fracture zone are marked as TB 1 —TB 4 . Scale bar, 10 nm. ( b ) Under tensile loading, the NW experiences elastic elongation as evidenced by the increase in spacing between TB 3 and TB 4 . Scale bar, 10 nm. ( c ) At the elastic strain of 6.8%, the Au NW breaks suddenly with a relatively flat fracture surface, typically encountered in brittle fracture. Scale bar, 10 nm. ( d , e ) Post-deformation fracture morphology of Au NWs at the two ends. A large de-twinned grain is found at both ends. Scale bar, 5 nm. ( f ) Full atomistic view and ( g ) cross-sectional view of Au NW with uniform twin distribution and λ =1.4 nm after fracture at 5.5% tensile strain by MD simulation. ( h ) Close-up view of the fracture region at the onset of yielding showing the homogeneous nucleation of dislocations indicated by vertical arrows, near surface facets but inside the NW. Atoms in perfect FCC crystal arrangement have been omitted for clarity. Full size image We examine the local shear strains computed at atomic-level from MD simulations to gain insight into the relationship between homogeneous nucleation, the de-twinning process and brittle-like fracture. Here, particular focus is placed on an ultra-twinned Au NW with λ =1.4 nm and a {111} microfaceted morphology ( Fig. 4 and Supplementary Movie 4 ). At the yield point, nucleation of dislocation loops on different slip planes is solely found inside the crystal ( Fig. 4a ). Notably the nucleation sites are primarily adjacent to surface facets (see inset of Fig. 4b ). At this stage of deformation, the average shear strain at a nucleation site is equal to 0.136±0.011, which agrees well with the ideal shear strain of 0.142 found theoretically by ab-initio simulations [27] for {111}<112> slip in Au. It can also be noticed that the yield strength of 5.5 GPa for <111> tension ( Supplementary Fig. S5 ) is generally higher than in experiments, which can be attributed to the strain rate effects inherent to MD simulations, the interatomic potential used, and the uncertainty in NW shape (see MD simulations method). However, it can be concluded that the yield strength of Au NWs with UDTs rises up to the ideal strength limit, thereby making homogeneous dislocation nucleation the rate-limiting process controlling fracture. As discussed later, we hypothesize that homogeneous nucleation in ultra-twinned Au NWs is induced by an instability comparable to that only found in perfect FCC crystals subjected to nanoindentation or shock loading [28] , [29] . Homogeneous dislocation nucleation is rapidly followed by shear localization and specimen necking, which are both accommodated by twin migration and de-twinning ( Fig. 4d and Supplementary Fig. S7 ). Here de-twinning arises from the atomic ledges formed at neighbouring TBs during homogeneous nucleation, and the shear localization when dislocations transmit through the TBs ( Fig. 4c–f ). While de-twinning promotes softening [14] and can partly enhance ductile plasticity, shear localization and necking accelerate the state of instability, which may partly explain the occurrence of both de-twinned tips and limited elongation in ultra-twinned Au NWs ( Fig. 4e ). 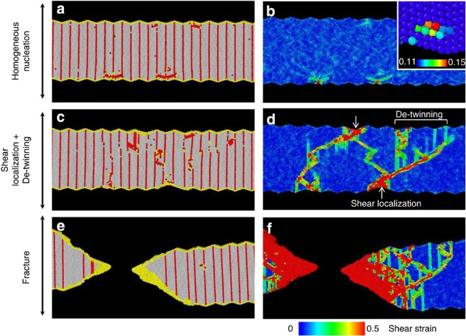Figure 4: Simulated deformation structure and shear strain in a brittle-like Au NW over the yielding process. The Au NW contains UDTs withλ=1.4 nm and {111} surface microfacets. (a,b) Homogenous nucleation, 5.2% strain. (c,d) Plastic shear localization and de-twinning, 5.6% tensile strain. (e,f) Fracture above 5.75% strain. Figure 4c also suggests that the absence of work-hardening in NWs with UDTs is related to the lack of dislocation blockage by TBs [5] and dislocation storage. The simulated fracture of a brittle-like NW with λ =0.7 nm ( Supplementary Fig. S7 and Supplementary Movie 5 ) further reveals that the local UDTs become largely unstructured in the fracture zone due to significant shear localization-induced necking, which confirms that this deformation mechanism becomes increasingly more important over de-twinning, as λ decreases to the minimum limit. Figure 4: Simulated deformation structure and shear strain in a brittle-like Au NW over the yielding process. The Au NW contains UDTs with λ =1.4 nm and {111} surface microfacets. ( a , b ) Homogenous nucleation, 5.2% strain. ( c , d ) Plastic shear localization and de-twinning, 5.6% tensile strain. ( e , f ) Fracture above 5.75% strain. Full size image Semibrittle fracture in Au NWs with bimodal twin structures A striking aspect is the strong dependence of fracture on λ in ultra-twinned Au NWs. Remarkably, ultra-twinned Au NWs with bimodal twin structures show a compromise between strength due to homogeneous slip, and some microplasticity via de-twinning and strain-hardening, leading to the semibrittle fracture ( Fig. 1c ). Further TEM evidence is shown in Fig. 5 where TBs of interest in the fracture zone are marked out in yellow colour. It is noticed that λ is not uniform along the axial direction in this specimen ( Fig. 5a ), and follows a bimodal twin distribution ( Supplementary Fig. S1b ). In Fig. 5b , plastic deformation starts in the region with the largest λ (between TB 3 and TB 7 with λ ~2.4–3.3 nm) in good agreement with past theoretical predictions [30] . As described above, dislocations and SFs are observed to nucleate directly inside the crystal ( Fig. 5b ); however, several partial dislocations are blocked by TBs (TB 3 and TB 6 in Fig. 5b ), which likely contributes to the apparent strain-hardening of the bimodal sample ( Fig. 1c ). Twinning partials causing de-twinning (shown in white reversed ‘T’ at TB 3 in Fig. 5b and TB 2 in Supplementary Fig. S8 ) are clearly visible because the Schmid factor for this type of slip is extremely low due to the TB orientation orthogonal to the NW axis. As deformation proceeds, shear localization promotes necking formation at the free surface (marked out with red-colour arrows in Fig. 5c ) after limited uniform plasticity. Propagation of SFs parallel to the twin plane accompanies necking ( Fig. 5c and Supplementary Fig. S8 ), and appears to soften the material in this region until failure. Also a tiny tip is visible in the fracture zone as a footprint of post-yielding plasticity from de-twinning ( Fig. 5d ). 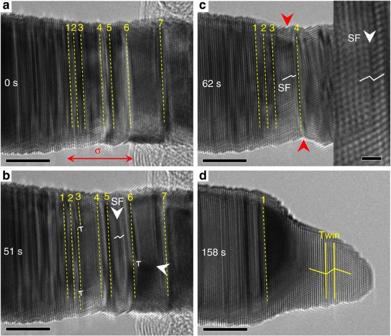Figure 5: Deformation and fracture in a semibrittle Au NWs with bimodal twin structures. (a) Pristine Au NW with a bimodal twin structure as marked out by dash lines in yellow from TB1to TB7. (b) As deformation proceeds, dislocations are observed to homogeneously nucleate in the segment with the largest twin thickness. The dislocations propagate and are blocked by the neighbouring TBs, causing strain-hardening. (c) Shear localization-induced necking formation under tensile loading, as marked out by the red arrows. Inset: Close-up on a partial dislocation with SF propagating along the radial direction from the neck, which softens this region and accelerates failure. (d) Fracture morphology of semibrittle fracture with de-twinned tips. Main scale bar, 5 nm; Inset scale bar inc, 1 nm. Figure 5: Deformation and fracture in a semibrittle Au NWs with bimodal twin structures. ( a ) Pristine Au NW with a bimodal twin structure as marked out by dash lines in yellow from TB 1 to TB 7 . ( b ) As deformation proceeds, dislocations are observed to homogeneously nucleate in the segment with the largest twin thickness. The dislocations propagate and are blocked by the neighbouring TBs, causing strain-hardening. ( c ) Shear localization-induced necking formation under tensile loading, as marked out by the red arrows. Inset: Close-up on a partial dislocation with SF propagating along the radial direction from the neck, which softens this region and accelerates failure. ( d ) Fracture morphology of semibrittle fracture with de-twinned tips. Main scale bar, 5 nm; Inset scale bar in c , 1 nm. Full size image This study provides strong evidence for a heterogeneous-to-homogeneous dislocation nucleation in ultra-twinned Au NWs below a critical twin size ( λ ≤2.8 nm). As significant slip activity was observed before failure, yielding in Au NWs with UDTs should be viewed at the atomic scale as being different from classical brittle fracture by atomic cleavage [31] . With UDTs, slip is confined in such a way that the elastic strain energy cannot be easily released by means of dislocation propagation [6] . Instead, homogeneous dislocation nucleation multiplies primarily near low-index surface facets, such as {111} microfacets, causing an avalanche of new dislocations that accelerates shear localization and necking. Therefore, Au NWs with bimodal twin structures show a composite behaviour between ultimate strength and a few percent of ductility, within a relatively narrow twin size distribution. In this case, the local increase in λ provides enough volume for dislocations to propagate and interact with neighbouring TBs in other areas of the NW, thereby explaining the emergence of strain-hardening and ductility via de-twinning [5] , [15] . Surprisingly, the ductile-to-brittle transition promoted by the heterogeneous-to-homogeneous dislocation nucleation with increasing twin densities, is totally opposite to the change from brittle fracture to ductile plasticity reported so far in nanotwinned ultrafine-grained Cu materials [11] , and recent experiments on single-crystalline Cu nanopillars and NWs with ultrathin twins [18] , [32] . The ultrafine-grained Cu containing nanotwins exhibits increasing softening and ductility with decreasing λ [11] , [12] , because deformation mediated by GBs are typically responsible for a transition from brittle fracture to extended ductility with decreasing λ [12] . Recent experiments on nanotwinned Cu nanopillars without GBs [32] have shown a brittle-to-ductile transition in samples loaded perpendicularly to TBs, as the TB spacing decreases below a critical value (~3-4 nm), in which the deformation was found to be dominated by the heterogeneous nucleation of dislocations from the intersections of TBs with the free surface. The brittle-to-ductile transition resulted from such heterogeneous nucleation of dislocations from the TBs/surface intersections, and shear band formation propagating across the samples [32] . This distinctive behaviour can possibly be understood by considering three factors. First, the stacking-fault energy curve being different between metals [33] , the stresses required to nucleate new dislocations from both heterogeneous and homogeneous nucleation is 2–3 times larger in Cu than Au [34] . However, the tensile strength previously measured in 50-nm nanotwinned Cu nanopillars (1.35 GPa) [32] is twice as small as that of our ultra-twinned Au at a comparable twin size ( λ =1.4 nm), which is indicative that the deformation mechanisms in Cu nanopillars with ultrathin twins are not related to homogeneous dislocation nucleation like Au NWs with UDTs. Second, the diameter of Au NWs in this study is the smallest ever reported in the literature for metallic NWs with UDTs. Past theoretical studies have shown that TBs exert a repulsive force on gliding dislocations due to image effects across the interface [30] , [35] . Such repulsive force increases linearly with 1 /λ , and the slope of this linear relationship was found to double with decreasing NW diameter from 25 to 8 nm (refs 30 , 36 ). Brittle-like fracture may therefore occur in ultra-twinned Au NWs with λ ≤2.8 nm because the theoretical strength limit is likely more rapidly attained than in larger NWs. This assumption is also supported by the fact that only softening due to heterogeneous dislocation nucleation from the TB-surface intersection was found in larger Cu nanopillars with ultrathin twins [32] . Third, the ideal strength limit in a metal has been shown to be dictated by instabilities in the acoustic phonon spectra [37] . In semiconductor crystalline NWs, phonon spectra and vibrational behaviour can be markedly influenced by the type of surface facets, such as {111} microfacets [38] . Surface effects on homogeneous dislocation nucleation are also manifest from our MD simulations ( Supplementary Fig. S6 ). Furthermore, past atomistic studies in circular metallic NWs have shown that the TB-surface intersections may have the largest atom vibration and higher stress concentration [36] , [39] . In metallic NWs, however, surface effects remain largely unexplored, primarily because characterizing the details of the surface structure at the atomic scale is extremely challenging experimentally. Nevertheless, the fact that ultra-twinned NWs in Cu and Au have been synthesized by different methods suggests that these NWs may have different surface structures and, therefore, different mechanical behaviour with increasing twin density. In conclusion, we report direct quantitative measurements on individual, ultrathin Au NWs with UDTs by in-situ tensile testing inside a TEM. These findings shed lights on a new regime of fracture in metallic NWs, and its physical mechanism, which can be controlled by modulating twin densities and therefore represents a new type of size effect distinct from sample size effects described previously. Furthermore, the conclusions of this study demonstrate the possibility of fabricating gold nanostructures with a desirable combination of ultrahigh strength and some ductility through optimization of the twin structure, which is of technological importance for micro-devices subjected to extreme stresses. In-situ experiments Two types of experiment were conducted. First, the Nanofactory TEM-scanning tunneling microscope (STM) platform with an AFM cantilever (App. Nano Inc.) serving as a force sensor was used to measure the stress–strain curves of Au NWs. The spring constant ( k ) of the cantilever was calibrated as 28 N m −1 . Then, a Nanofactory TEM-STM platform with a STM probe was used to study the deformation mechanism under in-situ HRTEM. All experiments were carried out inside a FEI Tecnai F30 field emission gun TEM. The NWs were attached to a piezo-controlled STM probe and then driven to approach the cantilever or the other STM probe. Finally, they were welded together by amorphous carbon deposition at the contact area via the illumination of low intensity electron beam. Subsequently, the NW was pulled back. The real-time images of sample elongation and the deflection (Δ d ) of cantilever were recorded by a CCD (charge-coupled device) camera at two frames per second. The tensile loading force ( F ) was directly calculated by timing the deflection Δ d by its spring constant k . The engineering stress was calculated by using the formula, where d is the NW diameter, and assuming that the NWs have a quasi-circular cross-section. The engineering strain was calculated by measuring the real-time length of the NWs from TEM images. More details on the in-situ experimental set-up can be found in our previous study [6] . Materials The synthesis of Au NWs was based on the method described in Wang et al . [40] Eighteen millilitres oleylamine (OAm) was heated to 60 °C under gentle N 2 flow. In another container, 44 mg HAuCl 4 · x H 2 O was dissolved in a mixture of 0.2 ml OAm and 2 ml hexane. The HAuCl 4 · x H 2 O solution was injected into the 60 °C OAm and held at the same temperature for 15 h without any disturbance such as magnetic stirring. After cooling to room temperature, 10 ml ethanol was added to precipitate the Au NWs. Au NWs with varied diameters can be made from different synthesis temperatures. Supplementary Fig. S9 shows the representative morphology of as-synthesized Au NWs with UDTs. Typically, the diameter of Au NWs presented in our study was uniform along the axial direction. Also, some variations in diameter were only observed at the two ends of the NWs. HRTEM study shows that the Au NWs are highly twinned ( Fig. 1a ). However, some of the high-density TBs in the TEM images will be invisible if the view zone slightly deviates from the [110] zone axis ( Supplementary Fig. S2 ). Au NWs were tilted to the [110] zone axis before tensile testing for the in-situ HRTEM study. Tensile loading was applied along the NW axis in the <111> direction until failure. For the TEM–AFM study, only Au NWs with uniform diameter and clean surface were chosen for the mechanical test. The NW ends were ‘glued’ to the AFM cantilever, and, therefore, did not significantly contribute to the deformation and strength measurements. Furthermore, all samples failing near the NW ends have been excluded in the mechanical data and fracture analysis. More than 20 samples were tested and about 40% were found to break with a brittle-like fracture. Au NWs with LDTs and no twins were created inside the TEM by using the cold welding technique. MD simulations MD simulations were performed using the software LAMMPS [41] with an embedded-atom-method potential for Au by Grochola et al . [42] We note that this potential was developed to simulate the growth and morphology of Au nanoparticles based on first-principles calculations, and, therefore, accurately predicts the SF and surface energies of this metal. Twelve realizations with uniform UDTs using different periodic lengths (68 and 270 nm), different twin densities (0.7≤λ≤5.6 nm) and different surface structures (perfectly circular and {111} microfaceted morphologies) were performed. [111]-oriented, periodically twinned NWs with a uniform λ were constructed by stacking platelet-like grains with a truncated octahedral shape made only by {111} surface facets. Owing to UDTs, this type of structure produced smooth sidewalls with atomic facets similar to those observed in experiments in Fig. 1b . Cylindrical NWs with same λ were also modelled with a circular cross-section in order to characterize the effect of surface morphology. Each twin plane was perpendicular to the NW axis, that is [111] crystallographic direction. Periodic boundary conditions were imposed along the NW axial direction, while the sides were kept free in all other directions. The diameter and periodic length were equal to 12 and 68 nm, respectively, for all wires. The time step was 2 fs. Before deformation, each model was relaxed for 40 ps under zero pressure using an isothermal–isobaric (constant number of particles N, constant pressure P, constant temperature T) ensemble with a Nose-Hoover thermostat at 300±2 K. Temperature was rescaled after 500 steps. The NW was deformed in tension by stretching the simulation box along the [111] direction at a constant engineering strain rate of 1 × 10 8 s −1 in the canonical (constant N, constant volume V, constant T) ensemble at the same temperature. Atomic-level snapshots of NW deformation were studied using the bond angle analysis and the local shear strain calculation in the atomic visualization software Ovito [43] . The Virial theorem and deformed atomic volume were used to calculate the axial stress in the NWs. Stress–strain calculations were based on the periodic lengths and average diameter, and did not take into account the local deformation due to necking. Error in strain calculations was limited because the simulations were performed at a constant engineering strain rate. However, caution was exercised in dealing with the stress values obtained after the onset of necking. In particular, deformations in brittle-like NWs were mostly elastic except for a localized plastic zone, as opposed to the behaviour of ductile NWs. It is, therefore, possible that larger elastic energy was released during fracture with the longer NWs, contributing to the length effect observed in Supplementary Fig. S5 . Moreover, it is noticed that the strength (5.5 GPa) of NWs with UDTs predicted in simulations is higher than in experiments. The strain rate effects inherent to MD simulations could be a factor. Another reason is that the interatomic potential used in our simulations could largely overestimates the ideal strength of {111}<112> slip in Au (1.73 GPa) compared with more accurate ab-initio simulations (1.42 GPa) (ref. 27 ). Also, the NW shape could influence the maximum stress predicted in MD simulation ( Supplementary Fig. S6 ). The {111} surface microfacets is revealed in Fig. 1b , but it could not be used to fully comprehend the three-dimensional shape of the NWs. So stress predictions from simulations could also be overestimated because very idealized models have been used. Thus, the ideal strength of 5.5 GPa predicted by our MD simulations should be viewed as an upper limit for the ideal strength of <111>-oriented Au crystals. How to cite this article: Wang, J. et al . Near-ideal theoretical strength in gold nanowires containing angstrom scale twins. Nat. Commun. 4:1742 doi: 10.1038/ncomms2768 (2013).